Auto-production of biosurfactants reverses the coffee ring effect in a bacterial system The deposition of material at the edge of evaporating droplets, known as the ‘coffee ring effect’, is caused by a radially outward capillary flow. This phenomenon is common to a wide array of systems including colloidal and bacterial systems. The role of surfactants in counteracting these coffee ring depositions is related to the occurrence of local vortices known as Marangoni eddies. Here we show that these swirling flows are universal, and not only lead to a uniform deposition of colloids but also occur in living bacterial systems. Experiments on Pseudomonas aeruginosa suggest that the auto-production of biosurfactants has an essential role in creating a homogeneous deposition of the bacteria upon drying. Moreover, at biologically relevant conditions, intricate time-dependent flows are observed in addition to the vortex regime, which are also effective in reversing the coffee ring effect at even lower surfactant concentrations. When the contact line of an evaporating droplet on a solid substrate is pinned, the surface tension sets up a capillary flow directed towards the edges. This capillary flow carries suspended matter to the edges of the droplet and results in deposition near the contact line. This process is commonly referred to as the ‘coffee ring effect’ [1] . Typically, the outward flow will be enhanced by an increase in the evaporative flux near the contact line [2] . However, there are several factors that can counteract this flow within the droplet, all of which derive from the occurrence of gradients in surface tension, known as Marangoni effects [3] . For example, thermal cooling near the contact line causes stresses, which counteract the outward capillary flow and a strong recirculating flow is predicted to occur [4] . However, temperature-driven Marangoni flows are rarely observed. As Hu and Larson [5] have shown, small quantities of contaminants result in significant Marangoni stresses that suppress these temperature-induced vortices. Surfactants can also impact significantly on the coffee ring effect as they have a dramatic effect on the surface tension gradients within a droplet. For insoluble surfactant systems, Van Nguyen and Stebe [6] , [7] demonstrated the occurrence of Marangoni–Bénard cells with an intricate pattern formation, due to the coupling between local temperature gradients and thermodynamic transitions at the surface. For soluble surfactants on the other hand, recent work qualitatively investigated the effect of SDS on the evaporation of aqueous drops. The compositional Marangoni stresses within these droplets created localized vortices, termed ‘Marangoni eddies’. These eddies have a dramatic effect on particulate deposition, giving a rather uniform deposition of material during evaporation [8] . Although this has received little or no attention so far, the coffee ring effect can also be observed in bacterial systems. This leads to very dense deposits of bacteria near the contact line. However, in the present work, using simple experiments of evaporating droplets containing live bacteria ( Pseudomonas aeruginosa ), no coffee ring depositions were observed. We will show that the presence of an auto-produced biosurfactant induces Marangoni stresses that reverse the outward capillary flow, leading to a homogeneous distribution of the bacteria upon drying. In contrast, a heterogeneous deposition of the bacteria, concentrated at the contact line, is obtained using a knock-out mutant that is unable to produce these biosurfactants. In addition to further investigate the role of surfactants on biological systems, while maintaining quantitative control of the surfactant concentration and properties, we performed a study on the role of exogeneously supplied non-ionic surfactants on the dynamics of eGFP-expressing Escherichia coli systems during drying. The experimental observations are compared with numerical calculations to rationalize the observed phenomena. Drying drops of P. aeruginosa show complex internal flows We found that when droplets of cultured P. aeruginosa were spotted on solid agar–agar plates, no coffee ring depositions were observed. Rather, a more uniform distribution of the bacteria was obtained. An example of such a spot, prepared using standard procedure, can be seen in Fig. 1b . Interestingly, when further experiments were carried out using a mutant, where the gene responsible for the production of biosurfactant (that is, rhamnolipid) was knocked out, significant deposition near the contact line was observed, as is shown in Fig. 1a . Moreover, the knock-out mutant did show a more homogenous deposition upon addition of exogenously supplied rhamnolipids and thus was able to overcome coffee ring depositions at the edge, similar to the wild-type. Our observations suggest that the mutant bacteria were subject to the capillary flow, whereas the wild-type bacteria gave a nearly uniform distribution of bacteria after drying due to the production of the biosurfactant rhamnolipid, which counteracted this flow. Our results show an improvement over previous reported attempts to obtain homogeneous depositions in droplets [8] , [9] . 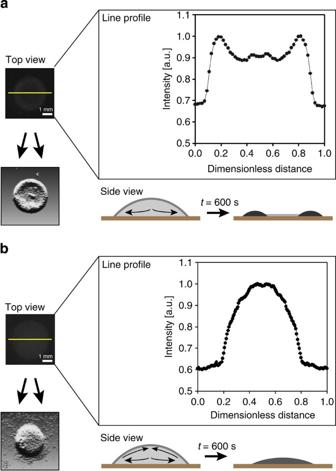Figure 1:P. aeruginosaproduces a biosurfactant that induces a Marangoni flow and inhibits the coffee ring effect. Droplets of liquid culture ofP. aeruginosaare spotted on solid agar–agar plates for a rhamnolipid production deficient mutant (a) and a wild-type (b). The mutant undergoes the capillary flow producing a coffee ring during drying, leading to bacteria being heaped up at the contact line. The wild-type gives a more uniform distribution of cells after drying due to the production of the biosurfactant rhamnolipid, which induces a Marangoni flow and inhibits the coffee ring effect. Intensity line profiles of the respective colonies are shown to indicate this phenomenon and statistical analysis confirms these findings (see Methods on image analysis). For both, a post-processed image of an example of a colony is shown, as a guide of the eye. The scale bar, 1 mm. Figure 1: P. aeruginosa produces a biosurfactant that induces a Marangoni flow and inhibits the coffee ring effect. Droplets of liquid culture of P. aeruginosa are spotted on solid agar–agar plates for a rhamnolipid production deficient mutant ( a ) and a wild-type ( b ). The mutant undergoes the capillary flow producing a coffee ring during drying, leading to bacteria being heaped up at the contact line. The wild-type gives a more uniform distribution of cells after drying due to the production of the biosurfactant rhamnolipid, which induces a Marangoni flow and inhibits the coffee ring effect. Intensity line profiles of the respective colonies are shown to indicate this phenomenon and statistical analysis confirms these findings (see Methods on image analysis). For both, a post-processed image of an example of a colony is shown, as a guide of the eye. The scale bar, 1 mm. Full size image To evaluate whether Marangoni flows formed the basis of the difference in the deposition patterns illustrated in Fig. 1 , we visualized GFP-labelled P. aeruginosa . When a droplet, containing bacteria in the stationary growth phase, was deposited on a microscopy slide and imaged using fast multi-focal microscopy, the flow patterns inside the drying droplet were observed to be complex and time dependent. For drying times >200 s, vortices were observed, similar to the Marangoni eddies observed by Still et al . [8] for the case of water droplets in the presence of SDS. Supplementary Movie 1 shows the swirling movement of an individual bacterium in the dense colony. Remarkably, for shorter drying times (<200 s), an intriguing time-dependent back and forth oscillatory flow was observed near the edge of the droplet. Fig. 2 shows the relative position of an individual bacterium with respect to the droplet edge, as function of time. An intriguing ‘ebb and flow’ dynamics is observed which has not yet been reported previously. P. aeruginosa bacteria auto-produce rhamnolipids, which are strong biosurfactants, and the concentration in the colonies typically amounts to 1 g l −1 in the stationary phase of growth [10] . The reported critical micelle concentration (CMC) for these biosurfactants is ~40 mg l −1 (ref. 11 ). Hence, the surfactant concentration in our droplets was about 25 times the CMC. At such concentrations well above the CMC, the occurrence of different concentration regimes (that is, the oscillatory flow and vortices) is somewhat surprising as the surface tension is expected to remain constant with concentration. 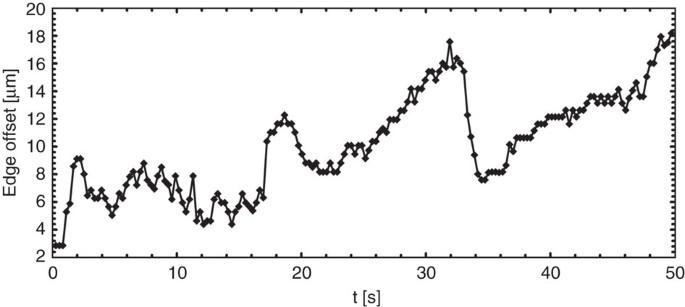Figure 2: Low concentrations of self-produced biosurfactants induce oscillatory flows in drying colonies. Plot of the time-dependent movement (horizontal axis, in seconds) of an individual bacterium ofP. aeruginosaand its offset to the edge of the droplet, that is, the relative distance between the droplet edge and the position of the suspended bacterium (vertical axis, in μm). A recurrent back and forth movement can be observed, reminiscent of the phenomenon of ‘ebb and flood’. The outward capillary flow in the droplet and the subsequent local concentration buildup of the biosurfactant at the edge creates an opposing Marangoni stress of equal strength that counteracts the coffee ring effect. Figure 2: Low concentrations of self-produced biosurfactants induce oscillatory flows in drying colonies. Plot of the time-dependent movement (horizontal axis, in seconds) of an individual bacterium of P. aeruginosa and its offset to the edge of the droplet, that is, the relative distance between the droplet edge and the position of the suspended bacterium (vertical axis, in μm). A recurrent back and forth movement can be observed, reminiscent of the phenomenon of ‘ebb and flood’. The outward capillary flow in the droplet and the subsequent local concentration buildup of the biosurfactant at the edge creates an opposing Marangoni stress of equal strength that counteracts the coffee ring effect. Full size image However, P. aeruginosa is not an ideal system to investigate these dynamics using confocal microscopy in detail due to its pathogenic nature and due to the high bacterial density under swarming conditions, which leads to a difficulty in imaging [12] . Additionally, to have more control over the surfactant type and its concentration in the droplet, non-biosurfactant producing E. coli was used to enable the systematic (more quantitative) study on the influence of exogeneously added surfactant, complementary to the rhamnolipid producing P. aeruginosa . These bacterial and other colloidal systems were studied to determine the role of surfactants in more detail and to explore the link with the different observed evaporation patterns. Different types of exogeneously supplied surfactants were used, including rhamnolipids. Vortices at high surfactant concentration Droplets containing eGFP-expressing E. coli bacteria in water were monitored during evaporation using confocal microscopy. The experiments were typically conducted using 10 μl droplets, placed on cover slips with small contact angles (≈6 ° ). It was carefully verified that the contact line of the droplets remained pinned during the time-window of our observations (see Methods on preparation of the sample). In Fig. 3a , for water droplets containing only a few bacteria, an outward flow from the centre of the droplet towards the edge was observed, causing the well-known contact line deposit [2] , [13] , [14] , [15] , [16] . In the presence of surfactants, the dynamics changed dramatically. A water droplet containing a high amount (1.25% w/v) of Triton X-100, a commonly used soluble non-ionic surfactant, showed vortices in a region near the edge of the droplet as is depicted in Fig. 3b . Near the bottom of the droplet, the bacteria were carried in the flow towards the droplet’s edge, but, once there, they were pulled upwards and inwards towards the centre of the droplet by this swirling flow. A detailed video showing these swirling flows via confocal microscopy is given as Supplementary Movie 2 . Over time, due to solvent evaporation, a self-concentration effect of the surfactant within the droplet occured, resulting in larger and stronger vortices. The vortex redistributed the bacteria in the droplet and counteracted the capillary flow. To verify that these observations were not influenced by the physical behaviour of the bacteria (for example, motility, chemotaxis) we fixed the bacteria using several approaches (see Methods on preparation of the tracer particles) and the experiments were repeated to confirm initial observations. Further confirmation of the generality of the observations was obtained by similar results with polystyrene beads ranging in size from 5 μm down to 200 nm. The predominant physical mechanism of our observations with bacteria is the same as for the inanimate colloidal systems. 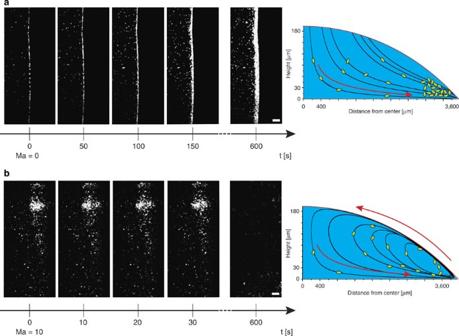Figure 3: The Marangoni flow induced by addition of surfactant overcomes the coffee ring effect. Capillary flow of eGFP-labelledE. colibacteria is observed in the absence (a) or presence of 1,25% w/v Triton X-100 (b). Marangoni numbers are calculated to be circa 0 and 10, respectively. In the absence of surfactant the capillary flow results in a narrow band of bacteria, which accumulates at the edge of the droplet, known as the coffee ring effect (a). Addition of Triton X-100, a non-ionic surfactant, induces a Marangoni flow opposing the coffee ring effect thus creating vortices, or swirling of the bacteria in the drop, depicted at the right. As a result, the bacteria are nearly uniformly deposited on the substrate upon drying. The scale bar, 30 μm and time is given in seconds. The schematics at the right are based on numerical integration of the velocity profiles calculated from the model discussed in the results. Figure 3: The Marangoni flow induced by addition of surfactant overcomes the coffee ring effect. Capillary flow of eGFP-labelled E. coli bacteria is observed in the absence ( a ) or presence of 1,25% w/v Triton X-100 ( b ). Marangoni numbers are calculated to be circa 0 and 10, respectively. In the absence of surfactant the capillary flow results in a narrow band of bacteria, which accumulates at the edge of the droplet, known as the coffee ring effect ( a ). Addition of Triton X-100, a non-ionic surfactant, induces a Marangoni flow opposing the coffee ring effect thus creating vortices, or swirling of the bacteria in the drop, depicted at the right. As a result, the bacteria are nearly uniformly deposited on the substrate upon drying. The scale bar, 30 μm and time is given in seconds. The schematics at the right are based on numerical integration of the velocity profiles calculated from the model discussed in the results. Full size image In order to investigate the effect of the surfactant, different concentrations and different types of non-ionic surface-active compounds were tested: Triton X-100, Tween 80, rhamnolipids and Triton X-114. Vortex formation is observed in all cases well above the CMC, at concentrations of 50, 500, 20 and 65 times the CMC of the used surfactant, respectively. Moreover, the solubility of Triton X-114 can be readily affected by temperature, as its cloud point is approximately at room temperature, 23 °C. For temperatures >23 °C, the surfactant solution starts to phase separate, resulting in a cloudy mixture [17] . This behaviour can be used to control the adsorption of the surfactant at the interface and hence also the Marangoni stresses. Indeed, measurements at slightly elevated temperatures (30±1 °C) prevented adsorption of the surfactant at the interface and no vortices were observed. By lowering the temperature, the vortices were reinstated. The observations of vortices emphasize the presence of an inward flow at the interface, directly opposing the radially outward capillary flow. Hu and Larson [4] , [5] showed that the Marangoni effect, created by a concentration gradient of surfactant molecules, is responsible for this phenomenon [4] , [5] . The spatial heterogeneity in surface concentration finds it origin in the same capillary flow that it opposes [18] , [19] , provided adsorption kinetics of the surfactant are not too fast. It is difficult to determine what the actual surfactant concentration gradients at the interface are, but our numerical simulations show that the Marangoni flow near the edge is much larger in strength than the outward capillary flow. The dimensionless Marangoni number (Ma) that characterizes the relative magnitude of Marangoni versus convective effects is defined as: where d σ /d Γ and d σ /d T are the change in surface tension ( σ ) with adsorbed amount of surfactant ( Γ ) and temperature ( T ), respectively, L is the characteristic length scale, η is the viscosity, D s is the surface diffusivity and α is the thermal diffusivity. For the case of Triton X-100 at 1.25% w/v, Ma ≈8.9 indicating that the regime in which the experiments were performed is dominated by Marangoni forces. Note that the Marangoni flow is also influenced by temperature gradients at the interface. Yet, this effect may be neglected in our case as Supplementary Table S1 shows that the evolution of the surface tension with temperature is much smaller than the evolution with concentration. Control experiments were also carried out with different droplet volumes (2–20 μl) and the obtained results all showed identical velocities, proving the independence of our observations of the vortices with droplet diameter. Oscillatory motion at low surfactant concentrations At a lower concentration of Triton X-100 (0.3% w/v) stationary vortices were no longer observed. Rather, reminiscent of the phenomenon of ebb and flow, the bacteria oscillated back and forth within the solution in close proximity to the pinned edge of the droplet, as shown in Fig. 4 . We know of no previous report describing such behaviour in literature. The bacteria were first convected outward, but before reaching the edge they moved back inwards. A diffuse front of the gathered bacteria formed, which underwent a time-dependent oscillatory motion parallel to the edge of the droplet ( Supplementary Movie 3 ). The timescale of these oscillations was independent of the droplet volume. These observations confirm that the addition of surfactant correlates with the strength of the Marangoni flow, which remains susceptible to variations in concentration, even in the regime above the CMC. For the lower concentration used (0.3% w/v), the opposing capillary and Marangoni flows are equal in strength (Ma ≈0.11), as sketched in Fig. 4 . 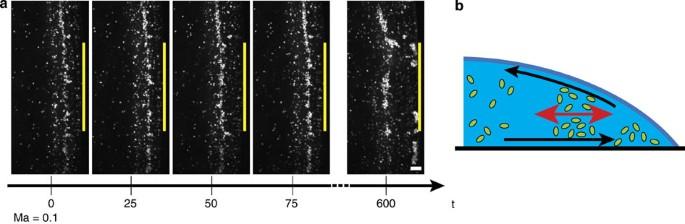Figure 4: Oscillatory movement of the bacterial front. A low concentration of surfactant induces a weaker Marangoni flow which is comparable in strength to the capillary flow. (a) Images of eGFP-labelledE. colibacteria showing a repetitive forward and backward movement of the collective front relative to the droplet edge (depicted in yellow). The backward movement is due to a Marangoni flow created by a low Triton X-100 concentration (0.3% w/v, Marangoni number of circa 0.1), which opposes the forward movement. (b) Schematic of the oscillatory back and forth movement (arrow in red) of the bacteria in the collective front (green). The capillary flow (bottom black arrow) results in accumulation of all solutes, both bacteria and surfactants, the last inducing the Marangoni flow (upper black arrow) opposing the coffee ring effect. The scale bar, 30 μm and time is given in seconds. Figure 4: Oscillatory movement of the bacterial front. A low concentration of surfactant induces a weaker Marangoni flow which is comparable in strength to the capillary flow. ( a ) Images of eGFP-labelled E. coli bacteria showing a repetitive forward and backward movement of the collective front relative to the droplet edge (depicted in yellow). The backward movement is due to a Marangoni flow created by a low Triton X-100 concentration (0.3% w/v, Marangoni number of circa 0.1), which opposes the forward movement. ( b ) Schematic of the oscillatory back and forth movement (arrow in red) of the bacteria in the collective front (green). The capillary flow (bottom black arrow) results in accumulation of all solutes, both bacteria and surfactants, the last inducing the Marangoni flow (upper black arrow) opposing the coffee ring effect. The scale bar, 30 μm and time is given in seconds. Full size image As time proceeds, the concentration of surfactant in the droplet increased and stationary vortices re-occured when the Marangoni flow gained in strength during the drying process. Trajectory analysis of the suspended bacteria in the microscopic images showed that for pure water, the velocity near the bottom of the plate during time interval t =(0–25) s equals 5.6±0.6 μm s −1 , whereas for water containing 0.3% w/v Triton X-100 the outward velocity is decreased to 4.6±0.3 μm s −1 , suggesting the presence of an inward flow. Moreover, this effect increases in strength during evaporation due to the aforementioned self-concentration effect. At t =(100–125) s, the velocity decreases further to 2.7±0.4 μm s −1 . As a consequence, the deposited pattern of bacteria on the substrate was nearly uniform, as shown in Fig. 3b , which bears a large similarity with our observations of the drying patterns of P. aeruginosa in Fig. 1b . No coffee ring pattern was observed for any of the surfactant concentrations studied here (0.1–1.5% w/v). This extends previous work where only minor inhibition of the coffee ring effect [9] or only a strong central accumulation [8] was obtained. Numerical simulations of the countercurrent flows To further analyse the observed phenomena, we investigated the influence of surfactants quantitatively starting from the model introduced by Hu and Larson [4] , [5] . The mechanisms that were taken into account are the capillary flow and the Marangoni effect. They are characterized using the Ma (Eq. (1)) and the bulk Péclet number (Pe): where u is the maximum velocity, L is the characteristic length scale and D is the bulk diffusivity. The required surfactant concentration to overcome the capillary flow could be readily calculated. The shear stress τ at the interface is given by: where r and z are the radial and vertical position within the droplet, respectively. The required Δ σ was calculated to be in the order of 0.001 mN m −1 . The predicted velocity profiles and trajectories ( Supplementary Fig. S1 ) reveal the presence of vortices at high surfactant concentrations, where the predicted velocities (±8.6 μm s −1 ) match the experimentally observed velocities (±9.1 μm s −1 ) in the vortex. Time-dependent oscillations and vortices At lower initial surfactant concentrations (0.3% w/v), we observed a periodic motion of the gathered bacterial front over time. 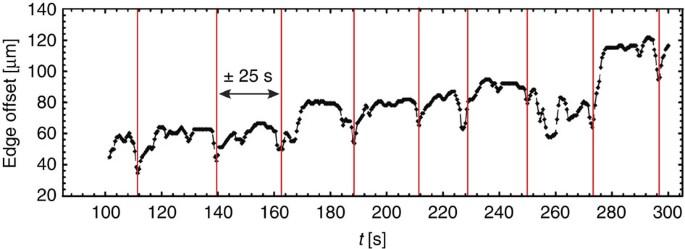Figure 5: Time-dependent influence of surfactant adsorption at the droplet interface. Plot of the time-dependent offset of the collective front of bacteria from the droplet edge. A periodic phenomenon is seen in the graph as there is a recurrent back and forth movement of the collective front. The characteristic frequency is approximately 0.04 Hz. Further, in time an increasing offset can be observed due to continuous thickening of the front, by accumulation of more bacteria, driven by capillary flow from the centre of the droplet. Figure 5 shows the bacterial position relative to the droplet edge in time, showing a recurrent timescale of ~25 s (or a characteristic frequency of ~0.04 Hz). We also observed a similar oscillatory behaviour with the same timescale for the vortices in the droplets with high surfactant concentrations (1.25% w/v, Supplementary Movie 2 ). These periodic phenomena suggest a dynamic competition between the outward capillary flow and the inward surfactant-induced Marangoni flow. Figure 5: Time-dependent influence of surfactant adsorption at the droplet interface. Plot of the time-dependent offset of the collective front of bacteria from the droplet edge. A periodic phenomenon is seen in the graph as there is a recurrent back and forth movement of the collective front. The characteristic frequency is approximately 0.04 Hz. Further, in time an increasing offset can be observed due to continuous thickening of the front, by accumulation of more bacteria, driven by capillary flow from the centre of the droplet. Full size image In all experiments, the surfactant concentration was above the CMC, resulting in a constant static surface tension value, independent of surfactant concentration. However, the complex interplay between the discussed flows within the droplet changes the concentration of the surfactant at the interface over time, for which the dynamic surface tension is the property to evaluate. To investigate if this dynamic surface tension is of the correct order of magnitude, an oscillating pendant drop module [20] , [21] , [22] , [23] , [24] was used. The response to a step change in interfacial area was probed on a system that was geometrically equivalent to the evaporating droplets. At low-step frequencies, diffusion is fast enough to replenish or remove surfactant upon dilation or compression, respectively, whereas at higher frequencies this is no longer the case [25] , [26] , [27] , [28] , [29] . This gives rise to an apparent surface ‘viscoelastic’ behaviour. Supplementary Fig. S2 shows the time evolution of the surface tension during the oscillating pendant drop method. This reveals that perturbations in adsorption of the surfactant—at the interface—level out over ~25 s, consistent with the previously observed frequency in the drop drying experiments of 0.04 Hz ( Fig. 5 ). In addition, a numerical calculation of the change of surfactant concentration and surface tension over time at the droplet interface confirmed our reported timescale (ca. 25 s) to be in the same order of magnitude ( Supplementary Fig. S3 ). This calculated time to saturate an initial clean interface upon addition of surfactant supports the idea that it is the process of diffusion, rather than demicellization and adsorption–desorption kinetics of the surfactant, which is crucial for the observed periodic behaviour [22] , [23] , [24] , [30] . The results suggest that the time dependence of the oscillations and vortices originates from a competition between the capillary and a Marangoni flow, which occurs due to an imbalance in surfactant concentration at the surface. The latter is opposite to the effect that creates the surface tension gradient (that is, the capillary flow), subsequently annihilating its own origin. The related timescale to rebuild the Marangoni effect is controlled by the kinetics of diffusion of the surfactant to the interface and competes with the timescale of the surface flow. The auto-production or exogenous addition of a soluble non-ionic (bio)surfactant induces complex flow patterns in a region near the edge of an evaporating droplet. This is due to the generation of a Marangoni flow, itself being created by a heterogeneous distribution of surfactant molecules along the interface by an outward capillary flow due to evaporation. The Marangoni stresses generated lead to full-blown vortices at high concentrations or after long drying times, but for lower concentrations, an oscillatory motion can be observed in the regime where capillary and Marangoni flow are equal in strength. Adding Triton X-114 as surfactant in the droplet and switching the temperature above and below the cloud point allows us to turn on and off the vortices and the oscillatory behaviour. In all cases upon addition of surfactants, it is the underlying physical phenomenon of the interplay between the capillary flow and the Marangoni stresses that leads to the observed macroscopic deposition patterns. Additionally, we found that both phenomena are time dependent, most probably controlled by the diffusion kinetics of the surfactant at the interface. Both colloidal and bacterial systems operate in a regime of dynamic equilibrium between the capillary and the Marangoni flow. Our observations show that even far above the CMC, an increase in the addition of surfactant still has a remarkable influence, in contrast to routine surface tension measurements. Changes in surface tension above the CMC indicate non-equilibrium conditions that exist in the system under study, as is shown by the transition from oscillatory behaviour to vortices. Experiments on a relevant biological sample illustrate how the self-produced surfactant in bacterial colonies leads them to distribute evenly upon drying. It is not clear whether this is essential in their survival, but the uniform deposition may have a biological advantage, as it fundamentally provides a mechanism enabling bacteria to spread over surfaces (for example, swarming) [31] , [32] , [33] , [34] . Often, these spreading mechanisms encountered are triggered by population densities reaching maximum limits, leading to a depletion of food sources for the cells present. The expansion over a surface to take in as much available resources may be a natural reaction to this unfavourable situation and hence a potential strategy used by biological systems. Our experiments indicate that biosurfactants have a significant role in the distribution of bacterial systems during drying, in general, in addition to the recently discovered role of self-produced surfactants in transport and movement processes [12] , [35] , [36] , [37] . Although our experiments were only conducted on P. aeruginosa , our conclusions are likely to be widely applicable and there are several other bacteria, which produce strong biosurfactants [35] , [38] . In conclusion, we prove that Marangoni stresses can generate sufficiently strong forces to drive both surface and bulk flows, either in swarming colonies or during drying of bacterial systems. Preparation of the substrate Single molecule clean cover slips were used for all imaging measurements to improve fluorescence signal-to-noise ratio and to obtain better wetting of the droplet on the silica substrate. Quantification of the resulting contact angle indicated an angle of 6 ° , opposed to non-cleaned cover slips that showed large contact angles of 40 ° (CAM-200, KSV Instruments, Finland). Cover slips were repeatedly rinsed with MilliQ water (0.055 μs cm −1 , Sartorius Stedim, France) and thermally treated for 24 h at 450 °C, followed by a UV-ozone reactor for 30 min. The surface roughness was checked with AFM measurements (SmartSPM 1000, AIST-NT, The Netherlands) and indicated that pinning of the droplet was not obtained by physical means, but rather chemically by the extreme hydrophilic substrate. Samples were imaged in air in non-contact mode with a drive frequency of 200–300 kHz. Silicon nitride oxide-sharpened tips were used. Imaging by confocal microscopy Fluorescent imaging was performed using a multi-beam confocal microscope (VisiTech, UK), equipped with an oil-immersion objective (× 20, 0.85 NA, Olympus, Japan) using 488 and 642 nm as excitation wavelengths. Full-frame (512 × 512 pixel resolution) images were acquired at 2 Hz. Temperature and relative humidity were controlled and monitored throughout all measurements (26±0.5 °C, 38±1% RH). Stable cooling and heating was provided for measurements with Triton X-114, combined with sufficient acclimatization of the system. Preparation of the sample The soluble non-ionic surfactants used were Triton X-100, Triton X-114 and Tween 80 and were purchased from Sigma-Aldrich (USA). Visualization of the contact line pinning was done in parallel experiments by staining the solution with the ATTO 647N dye (ATTO Tec, Germany), which allowed to spectrally separate the tracer signal (green) and the droplet edge (red), allowing careful control experiments and confirmation of pinning of the droplet edge. Measurements of surface tension Surface tension measurements were carried using the Wilhelmy plate method (KSV Instruments, Finland). A Teflon trough was used to allow temperature control. Necessary precautions were taken to limit contaminations and all solutions were allowed to stabilize overnight before measurements. Dynamic surface tension measurements were conducted using a custom-built improvement to the pendant drop system (KSV Instruments, Finland). Preparation of the tracer particles E. coli and P. aeruginosa were both used as biological tracers in this study for confocal microscopical investigation. E. coli K-12 (JM109 (DE3)) was transformed with eGFP/pRSET [39] by a standard protocol and spread on a luria broth plate with ampicillin (100 μg ml −1 ). After an overnight incubation at 37 °C, bacteria were picked up from a fluorescent colony and grown in 2 ml of luria broth (containing 100 μg ml −1 of ampicillin) at 25 °C (at 200 r.p.m.) for 6 h. The bacteria were subjected to the imaging after five subsequent washing steps by centrifugation, removal of the supernatant, and resuspension in Dulbecco’s phospate buffered saline (Invitrogen, USA). P. aeruginosa PA14 wild-type and its rhamnolipid production knock-out mutant were cultivated for swarming experiments according to the protocols in Fauvart et al . [12] Conditions for swarming were obtained by inoculating a spot of 2 μl of a P. aeruginosa culture, grown overnight in trypticase soy broth at 37 °C onto plates containing swarming medium (0.5% agar, 0.2% glucose, 1 mM MgSO 4 , 0.05 g casamino acids, 3.4 g Na 2 HPO 4 . 2H 2 O, 1.5 g KH 2 PO 4 , 0.25 g NaCl, pH 7). Incubation of plates was at 37 °C for 24 h, after which multiple volumes (ranging from 2–10 μl) were picked up of a proceeding swarming (tendril) tip and deposited on an agar-agar plate, left to dry for 10 min. These colonies were subsequently imaged using a plate reader (Flash and Go, IUL Instruments, Spain). For the microscopical visualisation, the harvested swarming bacteria and biosurfactants were deposited on a silica coverslip instead of an agar-agar plate. For these microscopic experiments, a fluorescently labelled mutant of P. aeruginosa PA14 was used by subcloning the Hind III- Ssp I Prh lA-GFP fragment from pYL122f in mini-CTX2 and subsequent electroporation to PA14, obtaining a chromosomal GFP fusion under control of the rhl A promotor. All experiments were repeated with dead bacteria, for which fresh cultures were treated with separate and combined exposure to 4% para-formaldehyde (Fisher Scientific, Belgium) and the antibiotic chloramphenicol (Roth Carl, Germany). Different exposure times (30, 120 and 240 min) to these chemicals or the combination hereof were tested. Viability tests of the bacteria were performed via cultivation and growth studies, to confirm the expected influence of the added chemicals. Additionally, different sized tracer particles were used. For the biological tracers, a measured outline of the bacteria (by the expression of fluorescent protein) of E. coli and P. aeruginosa were obtained using confocal microscopy (× 100 oil-immersion lens, 1.4 NA, Olympus, Japan) being 2.3 × 0.87 μm 2 and 1.7 × 0.45 μm 2 , respectively. Measurements with 200, 1,000, 2,000 and 5,000 nm sized polystyrene beads (Invitrogen, USA) confirmed our observations to be independent of the used tracer particles, which can be either biological or colloidal. Experiments with P. aeruginosa colonies on agar-agar plates were conducted in fivefold. Model simulation Flow profiles and streamlines were calculated using a numerical analysis method in MAPLE (version 14, Maplesoft, Canada). Adaptations to the model developed by Hu and Larson [4] , [5] comprise an additional contribution to the Marangoni effect due to surfactant concentration gradients: A numerical diffusion analysis of the surfactant concentration and surface tension evolution over time was performed in COMSOL Multiphysics (version 4.2, COMSOL Group, USA). A 1D diffusion equation was used, using parameters obtained from Stebe et al . [40] . Trajectory and image analysis Particle tracking was performed using custom-programmed software based on MATLAB (version 2011a, Mathworks Inc., USA). A Gaussian filter was applied to the images and trajectories were calculated using the nearest-neighbour algorithm. In Fig. 1 , for both type of colonies, mutant and wild-type species of P. aeruginosa , nine intensity line profiles were taken by rotation around the centre of the spotted colony. The average and variance of the corresponding bacterial population density, with respect to the position, was calculated and the average plot is shown. In case of the wild-type, a plateau can be seen in the centre of the colony due to inhibition of the coffee ring effect. This central plateau represents >40% of the droplet diameter, and for only 13.8% of these data points the variance significantly differs. These findings thus prove the flatness of the plateau and the nearly homogeneous deposition upon drying. For the non-producing biosurfactant mutant, two narrow peaks can be seen at each side of the droplet and these (too) represent 40% of the droplet diameter. Here the coffee ring effect occurs, as the capillary flow heaps up the bacteria at the edges and a small, lower central plateau is delineated. An enormous difference of 30% of the total height is seen between the valley and the peak and >39% of the data points from peak to peak statistically differ from the average (plateau) calculated. Again these findings confirm that in the case of mutant colonies it is the coffee ring effect that heaps up the bacteria at the edge, while for the wild-type P. aeruginosa this does not occur by a surfactant-induced Marangoni flow that inhibits the coffee ring effect. How to cite this article: Sempels, W. et al . Auto-production of biosurfactants reverses the coffee ring effect in a bacterial system. Nat. Commun. 4:1757 doi: 10.1038/ncomms2746 (2013).